Nanotechnology makes biomass electrolysis more energy efficient than water electrolysis The energetic convenience of electrolytic water splitting is limited by thermodynamics. Consequently, significant levels of hydrogen production can only be obtained with an electrical energy consumption exceeding 45 kWhkg -1 H 2 . Electrochemical reforming allows the overcoming of such thermodynamic limitations by replacing oxygen evolution with the oxidation of biomass-derived alcohols. Here we show that the use of an original anode material consisting of palladium nanoparticles deposited on to a three-dimensional architecture of titania nanotubes allows electrical energy savings up to 26.5 kWhkg -1 H 2 as compared with proton electrolyte membrane water electrolysis. A net energy analysis shows that for bio-ethanol with energy return of the invested energy larger than 5.1 (for example, cellulose), the electrochemical reforming energy balance is advantageous over proton electrolyte membrane water electrolysis. The exploitation of hydrogen in fuel cells has been widely advocated as the ideal solution for an energetically and environmentally sustainable future for transportation [1] , [2] . An essential part of such a solution will be the use of renewable energy resources (photovoltaics, wind, wave power and so on) in conjunction with water electrolysis to provide a ‘zero emission’ source of hydrogen [3] . Water electrolysis is a well-established commercial technology; nevertheless, its practical application for the mass production of hydrogen is still limited as it suffers from several major obstacles. The costly electrical energy consumption is certainly one of the major factors hampering the diffusion of electrolysis. This has been highlighted by the US Department of Energy (DOE). Indeed, in 2011, the DOE has pointed out that the electrical energy input to the electrolyser stack should drop from 45 to 43 kWhkg -1 H 2 by 2020 (ref. 4 ), while keeping constant the hydrogen production rate. Proton electrolyte membrane (PEM) electrolysers are at present the best-performing technology for the electrolytic production of hydrogen. This is because of the smaller ohmic (iR) losses as compared with the more traditional alkaline electrolysers [5] , [6] . Low iR losses allow PEM electrolysers to operate at current densities larger than 1 A cm −2 , thus producing useful quantities of hydrogen. Unfortunately, an inherent limitation to the diffusion of PEM electrolysers arises from the fact these devices employ acidic PEMs that require the use of expensive and rare platinum, ruthenium and iridium catalysts. Both alkaline and PEM electrolysers exploit water splitting, evolving hydrogen at the cathode and oxygen at the anode. The standard reaction potential for this process is 1.23 V, meaning that water splitting is a strongly uphill reaction. In practice, to get current densities in the range of 1 A cm −2 the cell potential usually ranges between 1.6 and 2 V (ref. 6 ). Considering 1.8 V as a reasonable average, we conclude that 68.3% of the energy input is consumed by thermodynamics, while kinetic factors account for only 31.7%. Replacing anodic oxygen evolution with the oxidation of much more readily oxidizable species leads to a significant reduction of the potential required to produce hydrogen. Following this strategy, compounds such as ammonia [7] , [8] , methanol [9] , ethanol [10] , [11] , [12] , [13] , glycerol [14] , [15] and urea [16] have been recently tested. These electrolytic processes that lead to the concomitant generation of chemicals at the anode and hydrogen at the cathode are often indicated as ‘electrochemical reforming’. Among these compounds, ethanol is certainly promising due to the possibility of production from the fermentation of biomass or steam reforming of cellulosic materials with reasonably low energy cost. The use of such compounds allows electrolysis at potentials <1 V, leading to electrical power savings as compared with conventional electrolytic water splitting. 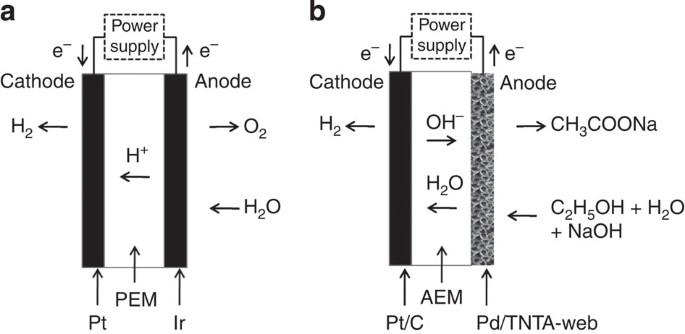Figure 1: Electrochemical reforming and water electrolysis comparison. Schematic of (a) PEM water electrolysis and (b) alkaline electrolyte membrane electrochemical reforming. Figure 1 shows schematically the difference between a state-of-the-art PEM electrolyser and an alcohol electrolyser. Figure 1: Electrochemical reforming and water electrolysis comparison. Schematic of ( a ) PEM water electrolysis and ( b ) alkaline electrolyte membrane electrochemical reforming. Full size image Equations (1, 2, 3) describe the anode, cathode and overall electrochemical-reforming reactions, respectively. While promising, these approaches suffer the limitation of delivering current densities well below 1 A cm −2 , and as such are unpractical for technological exploitation. Here we propose to overcome such limitations using three-dimensional (3D) nanostructured TiO 2 nanotube arrays (TNTA-web) as a support for Pd nanoparticles (NPs) (Pd/TNTA-web). The combination of Pd and TiO 2 nanotubes on flat surfaces has been recently shown to be effective for alcohol electro-oxidation [17] . The novelty of the approach consists in the fact that the TNTAs are prepared by the anodization of a Ti fibre web support rather than a titanium foil [17] . The system therefore does not rely on high surface area carbon supports, as previously reported for TiO 2 nanotube electrodes [18] , to obtain high Pd dispersion. In addition, no binder and/or ionomer are required to assemble the electrodes, allowing good mechanical stability and high utilization of the active phase. Here we demonstrate that electrochemical reforming can occur at current densities comparable to that of state-of-the-art PEM water electrolysis. Furthermore, we report for the first time a net energy analysis of hydrogen production by bio-ethanol electrochemical reforming. Particularly, we define the energy cost break-even point, expressed in terms of the energy return of the invested energy (EROI) [19] of bio-ethanol production, at which electrochemical reforming becomes more energy efficient than water electrolysis. 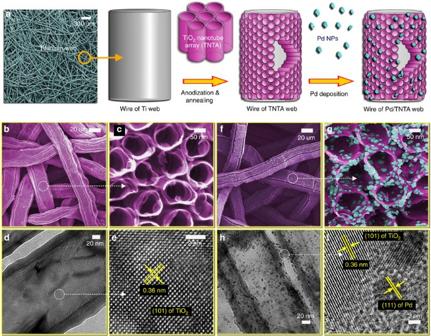Figure 2: Anode architecture schematics and electron microscopy characterization. (a) Scheme of the Pd/TNTA-web electrode preparation process (scale bar=300 μm). SEM (b, scale bar=20 μm;c, scale bar=50 nm), TEM (d, scale bar=20 nm) and HRTEM (e, scale bar=2 nm) images of the bare 3D TNTA electrode support and SEM (f, scale bar=20 μm;g, scale bar=50 nm), TEM (h, scale bar=20 nm) and HRTEM (i, scale bar=2 nm) images of the electrode after loading with 1.7 mg cm−2of Pd NPs. Characterization of anode material Figure 2a schematically shows the approach used for anode electrode fabrication. A commercial titanium non-woven sintered web support (thickness 0.5 mm, average fibre diameter 20 μm, 73% porosity) is used to confer the 3D structure to the system (shown in Fig. 2a ). This material has an open fibrous structure that allows for fast mass transport in the liquid phase. Figure 2: Anode architecture schematics and electron microscopy characterization. ( a ) Scheme of the Pd/TNTA-web electrode preparation process (scale bar=300 μm). SEM ( b , scale bar=20 μm; c , scale bar=50 nm), TEM ( d , scale bar=20 nm) and HRTEM ( e , scale bar=2 nm) images of the bare 3D TNTA electrode support and SEM ( f , scale bar=20 μm; g , scale bar=50 nm), TEM ( h , scale bar=20 nm) and HRTEM ( i , scale bar=2 nm) images of the electrode after loading with 1.7 mg cm −2 of Pd NPs. Full size image The synthesis consists of an anodization of the substrate performed in a fluoride-containing medium [20] (see Methods section). The result of this process is the formation of a finely distributed TNTA that completely covers the surface of the titanium fibres. Anodization is followed by an annealing step at 400 °C that increases the crystallinity and transforms the TiO 2 into the anatase phase. X-ray diffraction measurements confirm the presence of anatase after annealing [17] ( Supplementary Fig. 1 ). Palladium NPs are deposited on to the TNTA-web support using a chemical deposition procedure followed by reduction with NaBH 4 . Using this procedure electrodes with a Pd loading of 1.7 mg cm −2 were prepared. Figure 2b–i shows the field emission scanning electron microscopy (SEM)and the high-resolution transmission electron microscopy (HRTEM) characterization of the TNTA-web support and the Pd/TNTA-web electrodes. Figure 2b–d shows clearly the morphology of the TNTA. The individual nanotubes have an inner diameter of 100 nm with a wall thickness of ca. 10 nm and an average tube length of around 2.0 μm. Notably, the nanotube array covers homogeneously the entire surface of each of the titanium fibres of the web electrode. A high-resolution image of a single nanotube taken along the 101 zone axis of anatase shows a distance among the planes of 0.35 nm, in agreement with the reported data for the anatase unit cell size ( Fig. 2e ). A low-magnification field emission SEM micrograph ( Fig. 2f ) of the TNTA-web electrode after palladium addition does not show significant changes to the microstructure of the anodized/annealed electrode. At higher magnification ( Fig. 2g ), supported Pd NPs can be seen on the TNTA surface that has a bimodal size distribution. The Pd particles accumulated around the opening of the nanotubes have an average particle size of ca. 13 nm. A low-magnification TEM image ( Fig. 2h ) shows that particles are also present along the entire length of the nanotube walls, both outside and inside the nanotubes. Interestingly, the average size of Pd particles deposited along the inside of the nanotubes showed a smaller size (6–7 nm) as compared with the particles at the surface. An HRTEM image of the supported Pd NPs shows both the planes of anatase and the plane of metallic Pd ( Fig. 2i ). Palladium oxidation state has been investigated by X-ray photoelectron spectroscopy. Spectra reveald that both bare metal and oxides were present at the surface ( Supplementary Fig. 2 ). The electrochemical active surface area of Pd has been estimated by cyclic voltammetry (CV) in 2 M KOH using the charge associated with the reduction peak of the first monolayer of PdO (conventionally taken as that formed at 1.45 V versus reversible hydrogen electrode (RHE)) and was determined to be 45.9 m 2 g −1 Pd (ref. 21 ). Electrochemical-reforming experiments The Pd/TNTA-web electrode was employed as the anode in a PEM-type electrolyser ( Supplementary Fig. 3 ), equipped with an anion exchange membrane (Tokuyama A201) and a Pt/C on carbon cloth cathode (0.3 mg Pt cm −2 ). Parameters for electrolysis experiments are listed in Table 1 . An aqueous electrolyte consisting of 2 M renewable alcohol and 2 M NaOH was fed to the anode. No liquid was passed through the cathode compartment. Electrolysis polarization curves were obtained in the potential range from 0 to 1.0 V at 10 mV s −1 scan speed. Cell temperature was regulated between 25, 50 and 80 °C. 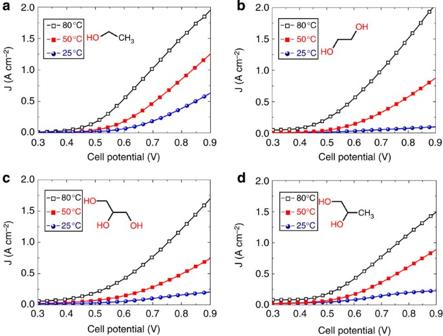Figure 3: Electrochemical reforming of alcohols with Pd on 3D Titania Nanotube Architecture. Polarization curves for 2 M NaOH water solutions of (a) 2 M ethanol; (b) 2 M ethylene glycol; (c) 2 M glycerol; and (d) 2 M 1,2-propandiol. Figure 3a shows typical electrolyser polarization curves obtained at 25, 50 and 80 °C with 2 M ethanol. Figure 3a shows that at 80 °C the output current density at a cell potential of 0.9 V was 1.95 A cm −2 , more than three times that observed at the same voltage at 25 °C (0.51 A cm −2 ). This behaviour can be ascribed to the enhanced kinetics of ethanol electro-oxidation with increasing temperature [22] . Interestingly, no mass transport limitation can be observed, even at the highest current densities. Indeed a productive electrolysis system needs to be operated at elevated current densities to deliver useful quantities of hydrogen. Such high current densities obtained in the alcohol electrolyser result from a combination of the unique open 3D structure of the anode electrode and the very high electrochemical active surface area of the supported Pd NPs, thus promoting very fast kinetics for alcohol oxidation. Indeed the current densities obtained are comparable to the best state-of-the-art PEM water electrolysers ( Table 1 ). Analysis of anode exhausts (HPLC, 13 C NMR) confirmed that sodium acetate was the sole product of ethanol oxidation as expected from a Pd-based electrocatalyst in alkaline media [23] . As expected, at the cell working potentials (<1 V) no oxygen evolution was detected. Table 1 Comparison of electrolyser performance*. Full size table Figure 3: Electrochemical reforming of alcohols with Pd on 3D Titania Nanotube Architecture. Polarization curves for 2 M NaOH water solutions of ( a ) 2 M ethanol; ( b ) 2 M ethylene glycol; ( c ) 2 M glycerol; and ( d ) 2 M 1,2-propandiol. Full size image From Table 1 data we can calculate that the use of ethanol ( 18.5 kWhkg -1 H 2 ) results in an electrical energy saving of 26.5 kWhkg -1 H 2 as compared with that reported by the DOE for PEM electrolyser stacks as of 2011 ( 45 kWhkg -1 H 2 ). The oxidation of other biomass-derived alcohols can also be considered for hydrogen production. Figure 3b–d compares the polarization curves obtained in the alcohol electrolyser with glycerol, ethylene glycol and 1,2-propandiol. We can see that in all cases the Pd/TNTA-web anode exhibits excellent activity and high output current densities. Table 2 shows that the energy consumption for H 2 production for all alcohols is in the range of 18.49– 20.63 kWhkg -1 H 2 . Table 2 Comparison of electrical energy input of the electrolyser fed with different renewable alcohols*. Full size table One may now consider whether from an overall energetic point of view the exploitation of ethanol in electrolysis is actually worthy of consideration. According to the calculations reported in Supplementary Note 1 , 11.4 kg of ethanol and 9.9 kg of NaOH are required to produce 1 kg of hydrogen. A recent of investigation of the ‘cradle to gate’ life cycle assessment (LCA) determined the NaOH energy cost to be 0.97 kWh kg −1 NaOH (ref. 24 ), which can be used to calculate an alkali-related energy expenditure of 9.7 kWh per kilogram of produced H 2 . Consequently, a net energy saving for H 2 production with respect to water electrolysis will be achieved if the cost of ethanol contributes <16.8 kWh per kilogram of produced H 2 . This is the case when the ethanol energy cost is <1.46 kWh kg −1 EtOH . The assessment of bio-ethanol net energy cost is usually expressed in terms of the EROI, namely, the ratio between: (i) the output energy from ethanol and (ii) the energy input required for its production. According to the DOE the output energy density for ethanol is 7.4 kWh kg −1 EtOH (ref. 25 ). On such a basis we can conclude that a bio-ethanol EROI larger than 5.1 is required to obtain a net energy saving with respect to current water electrolysis technology. The DOE target for electrolyser stack electric energy input for 2020 (ref. 4 ), 43 kWhkg -1 H 2 , is instead met for a bio-ethanol EROI larger than 5.3. Hence, hydrogen production by electrolysis of bio-ethanol will be energetically convenient depending on the source of the alcohol, for example, using sugarcane that is commonly reported to have an EROI of 8 and higher [26] , [27] and from cellulose with an EROI potentially up to 35 depending on the production methods [28] . It is worth mentioning that cellulose ethanol is particularly appealing as it can be obtained from the steam reforming of lignin. Lignin can be obtained even from spontaneously growing plants in lands not dedicated to agriculture, avoiding competition with the food chain supply [28] . The use of different bio-derived alcohols not only increases the versatility of the electrolysis process for H 2 generation, but also leads to the generation of valuable chemicals from the large variety of products that can be obtained by the electro-oxidation of such polyalcohols (for example, lactate, glycolate, oxalate, glycerate and tartronate salts; Supplementary Table 1 ). In conclusion, electrolysers operating with biomass-derived alcohols show the hydrogen production levels to be as high as the best-performing conventional water PEM electrolysers, providing at the same time net energy savings. Electrochemical reforming offers also the possibility to produce hydrogen at high pressure, eventually directly at 700 bar, the target for automotive applications [29] virtually eliminating energy-costly multistage compression. This is possible because no oxygen is evolved, reducing the risk of explosion from mixing with hydrogen. This would be impossible with current PEM electrolyser technologies as they cannot prevent completely the intermixing of oxygen and hydrogen, limiting pressurization to around 30 bar (ref. 6 ). Furthermore, partial oxidation of bio-alcohols leads to the formation of valuable by-products. As a consequence, we can hypothesize the exploitation of alcohol electrolysis as an essential component of the ‘biorefinery’ offering processes capable of producing both chemicals and hydrogen that can be used both as energy vector and reactant. Anode synthesis TNTAs were fabricated on the titanium non-woven web support surface by a combination of electrochemical polishing, anodization and annealing steps as follows: 1 Electrochemical polishing: After pre-washing the titanium non-woven web support with deionized water and acetone, an electrochemical polishing treatment was undertaken using a two-electrode cell, in which a titanium sheet (2.5 × 2.5 cm size) was used as the cathode electrode and the titanium non-woven web disk (1 cm 2 ) was the anode electrode (the distance between the cathode and anode electrodes was set at 2 cm). The electrolyte was 95 wt% acetic acid+5 wt% HClO 4 . The electrochemical polishing treatment was carried out at 60 V for 10 s at room temperature. 2 Electrochemical anodization: The electrochemical anodization was performed in the same two-electrode cell used for the electrochemical polishing treatment. The electrolyte in this case was 0.5 wt% NH 4 F and 99.5 wt% ethylene glycol, and the electrochemical anodization potential was set at 60 V for 60 min at room temperature. 3 Annealing: The anodized electrode was then annealed by heating to 400 °C (10 °C min −1 ) in air for 30 min. Palladium NPs were loaded on to the TNTA support using the following chemical deposition and reduction method: 1 A volume of 0.2 ml of a solution containing 0.3 g PdCl 2 , 0.7 ml HCl (37%) and 1 ml ethylene glycol in 50 ml of water was added drop-wise to the surface of the TNTA substrate (1 cm 2 disk). 2 The impregnated disk was then dried in an air atmosphere oven at 80 °C. 3 Steps 1 and 2 were then repeated until the desired quantity of Pd precursor loading was obtained. 4 The sample was then reduced in an ice cold aqueous NaBH 4 (0.1 wt%) solution for 12 h. 5 After reduction, the sample was washed thoroughly in deionized water and dried at 60 °C until constant weight. The Pd content of the electrode was assessed by removing a small piece and dissolving in hot concentrated HCl. After dilution the Pd content of this solution was determined by inductively coupled plasma mass spectrometry (ICP-MS) analysis. Material characterization The Pd content of the Pd/TNTA-web anode was determined by ICP-MS as follows. After testing, a weighted piece of the electrode was dissolved in hot concentrated HCl. After dilution the Pd content of this solution was determined by ICP-MS analysis with a quadrupole ELAN DRC-e spectrometer (PerkinElmer SCIEX, Concord, Ontario, Canada). TEM images were performed on a Philips CM12 microscope operating at 100 kV. The microscope was equipped with an EDS energy-dispersive microanalysis system. SEM was performed on a HITACHI S4800 microscope operating at 15 kV. HRTEM images were recorded with a Zeiss Libra 200 FE TEM equipped with a double tilt goniometer at 200 kV and FEI Tecnai-F30 microscope that was operated at 300 kV. X-ray diffraction patterns were acquired at room temperature with a PANalytical X’PERT PRO diffractometer, employing CuKα radiation ( λ =1.54187 Å) and a parabolic MPD mirror. The spectra were acquired in the 2 θ range from 20° to 80°. X-ray photoelectron spectroscopy measurements were performed with a PHI Quantum 2000 XPS system (Physical Electronics Inc., USA) using Al Kα (1486.6 eV) radiation to determine the composition of the as deposited Pd/TNTA-web electrode. The base pressure in the analysis chamber was of the order of 5 × 10 −8 Torr during data collection. The invariance of the peak shapes and widths at the beginning and at the end of the analyses ensured absence of differential charging. Analyses of the peaks were performed with the software provided by PHI Quantum, the binding energy values are quoted with a precision of ±0.15 eV and the atomic percentage with a precision of ±10%. CV for the electrochemically active area measurements were performed with a Princeton 2273A potentiostat/galvanostat, using a three-electrode arrangement with a saturated calomel reference electrode and a platinum foil (25 mm × 25 mm × 0.1 mm) as counter electrode. No iR-drop compensation was applied to any of the performed experiments. The potential scale of the CV curves was then converted to the RHE scale. The experiments have been conducted in 2 M aqueous KOH (Sigma-Aldrich 99.8%). All the solutions were prepared with Millipore water (18 Mωcm) provided by a Milli-Q labo apparatus (Nihon Millipore Ltd). Solutions were deaerated by bubbling high-purity N 2 before measurements. Electrochemical-reforming experiments The electrolysis test cell hardware was purchased from Scribner-Associates (USA) with a 25-cm 2 fuel cell fixture, which was modified in our laboratory with titanium end plates to tolerate the alkaline conditions. The cell temperature was regulated using a Scribner 850e fuel cell test station. The membrane electrode assembly (MEA) was fabricated by mechanically pressing together the anode (1 cm 2 Pd/TNTA-web), cathode (1 cm 2 Pt/C on carbon cloth) and a Tokuyama A201 alkaline exchange membrane. The cathode was prepared by coating an ink containing Pt/C 40 wt% (Aldrich) and nafion binder on to carbon cloth to give a Pt loading of 0.3 mg cm −2 . Electrolysis cell performance was determined using an ARBIN BT-2000 5A 4 channels instrument. The aqueous fuel solution (2 M NaOH and 2 M alcohol) was delivered to the anode compartment at 4 ml min −1 flow speed. The cell temperature was regulated at 25, 50 and 80 °C. The electrolysis cell was also run in water electrolysis mode with 2 M NaOH as electrolyte. The electrolysis cell was also used to determine the product distribution obtained after electrolysis of solutions of various alcohols. In each experiment 20 ml of a 1-M alcohol and 2-M NaOH solution was circulated through the anode compartment of the cell. The cell was heated to 50 °C and a constant electrolysis current was applied at 300 mA cm −2 and the cell voltage was monitored. The run was stopped when the cell voltage reached 1.1 V. The anode solution was then analysed by a combination of HPLC and 13 C NMR to determine the product distribution according to the methods described in Supplementary Method . How to cite this article: Chen, Y. X. et al . Nanotechnology makes biomass electrolysis more energy efficient than water electrolysis. Nat. Commun. 5:4036 doi: 10.1038/ncomms5036 (2014).